Müller cells separate between wavelengths to improve day vision with minimal effect upon night vision Vision starts with the absorption of light by the retinal photoreceptors—cones and rods. However, due to the ‘inverted’ structure of the retina, the incident light must propagate through reflecting and scattering cellular layers before reaching the photoreceptors. It has been recently suggested that Müller cells function as optical fibres in the retina, transferring light illuminating the retinal surface onto the cone photoreceptors. Here we show that Müller cells are wavelength-dependent wave-guides, concentrating the green-red part of the visible spectrum onto cones and allowing the blue-purple part to leak onto nearby rods. This phenomenon is observed in the isolated retina and explained by a computational model, for the guinea pig and the human parafoveal retina. Therefore, light propagation by Müller cells through the retina can be considered as an integral part of the first step in the visual process, increasing photon absorption by cones while minimally affecting rod-mediated vision. The primary event of vision is the projection of light by the optical system of the eye onto the proximal surface of the retina [1] . However, the mammalian retina and the peripheral retina of humans and primates are organized in a seemingly reverse order with respect to the light path. This arrangement places the photoreceptors, responsible for light absorption [2] , [3] , as the last cells in the path of light, rather than the first [4] , [5] . Therefore, the incident light must propagate through five reflecting and scattering layers of cell bodies and neural processes before reaching the photoreceptors. This ‘inverted’ retinal structure is expected to cause blurring of the image and reduction in the photon flux reaching the photoreceptors, thus reducing their sensitivity [6] , [7] , [8] , [9] . It has been recently reported that retinal Müller cells act as light guides serving to transfer light across the retina, from the vitreo-retinal border towards the photoreceptors [10] , [11] , [12] . However, the basic question remains: How does light propagation via Müller cells through the neuronal layers of the retina affect vision? A single Müller cell collects light at the vitreo-retinal surface from an extended retinal region, and guides it onto one coupled cone, located at its distal end [13] ( Fig. 1a ). Since the proximal, receiving end of the Müller cell is wide, compared with its distal part, and also covers ~15 rods surrounding the central cone ( Fig. 1a ), light concentration into the cone is expected to reduce the photon flux reaching the rods and thus impede rod-mediated vision, crucial for dark conditions [14] . On the other hand, if light guiding onto cones is ineffective, cone-mediated vision, crucial for day-time conditions, will suffer from a substantial loss of sensitivity due to light scattering by the neuronal retina. Can this cost-benefit optimization problem between day vision and night vision be solved, without significantly impeding one or the other? 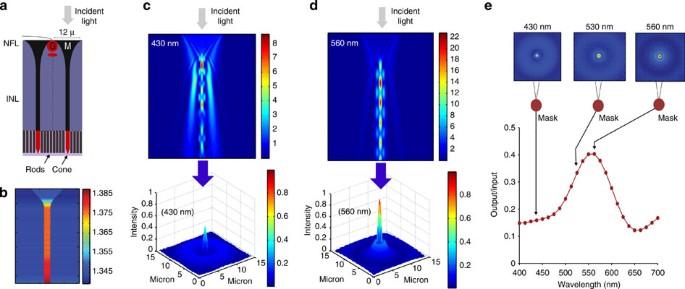Figure 1: Simulation of light guiding by human Müller cells. (a) Schematic representation of Müller cells (M) and photoreceptors organization in the human parafoveal retina. Müller cells' (in black) proximal cup-like funnel of ~12 μm in diameter, covers ~15 rods in addition to the central cone. Nerve fibre layer (NFL), and inner nuclear layer (INL) are outlined. (b) A data cube of 1,000 × 256 × 256 grid containing a Müller cell (of 130 μm length) and its surrounding tissue was reconstructed, based upon measured indices of refraction profile (scale on the right). (c,d) Simulation of light passing through a single Müller cell (top) and the corresponding distribution at the distal part of the cell (bottom), for an incident light of 430 nm (blue) and 560 nm (green–yellow). Light concentration into the centre (cone’s receptive field) is higher for the green than for the blue. (e) The transmitted spectrum into the central cone is calculated by summing the pixels inside the Müller cell’s area, and averaged over the last longitudinal intensity cycle. The peak transmission is at 560 nm, corresponding for the green-yellow part of the visible spectrum. Figure 1: Simulation of light guiding by human Müller cells. ( a ) Schematic representation of Müller cells (M) and photoreceptors organization in the human parafoveal retina. Müller cells' (in black) proximal cup-like funnel of ~12 μm in diameter, covers ~15 rods in addition to the central cone. Nerve fibre layer (NFL), and inner nuclear layer (INL) are outlined. ( b ) A data cube of 1,000 × 256 × 256 grid containing a Müller cell (of 130 μm length) and its surrounding tissue was reconstructed, based upon measured indices of refraction profile (scale on the right). ( c , d ) Simulation of light passing through a single Müller cell (top) and the corresponding distribution at the distal part of the cell (bottom), for an incident light of 430 nm (blue) and 560 nm (green–yellow). Light concentration into the centre (cone’s receptive field) is higher for the green than for the blue. ( e ) The transmitted spectrum into the central cone is calculated by summing the pixels inside the Müller cell’s area, and averaged over the last longitudinal intensity cycle. The peak transmission is at 560 nm, corresponding for the green-yellow part of the visible spectrum. Full size image Here we address these questions by computational modelling and experimental imaging methods. As a first step, we use a computational optical model to analyse light-guiding properties of Müller cells in the human parafoveal retina, and show that human Müller cells separate white light according to its wavelengths; medium- and long-wavelength light is concentrated onto cones and short-wavelength light leaks to illuminate nearby rods. Next, we show similar theoretical calculations for the guinea pig Müller cells and describe imaging experiments in the isolated guinea pig retina, to find remarkable agreement between the experimental results and the computational model. These findings are consistent with the hypothesis that the wave guiding properties of Müller cells are wavelength-dependent in a manner that improves cone-mediated vision while minimally impeding rod-mediated vision. Computational analysis of Müller cells’ light propagation As a first step in addressing the above question, we performed light propagation simulation for monochromatic light through the peripheral human retina. Using previously measured refractive index profile, obtained by phase microscopy measurements of human retinas [10] , we reconstructed a 1,000 × 256 × 256 data-cube grid, which contains a Müller cell and its vicinity in the human parafoveal retina [15] , [16] ( Fig. 1b and Supplementary Fig. 1 ). In order to calculate light propagation through the Müller data-cube, we have developed [11] and applied a known algorithm, the fast Fourier transform beam propagation method (FFT BPM) [17] , [18] , [19] , [20] , [21] . This is a direct three-dimensional (3D) numerical solution of the wave equation, also known as the scalar Helmholtz equation [22] , [23] : Here is the light propagating field and , where z is the propagation direction (across the retina), k =2π/λ, where λ is the wavelength of light, is the refractive index profile of the retina, and ∇ 2 =∂ 2 /∂ x 2 +∂ 2 /∂ x 2 +∂ 2 /∂ x 2 is the 3D derivative, the Laplacian (see Methods). An initial light distribution entering the cell was taken as a diffraction pattern from the eye’s pupil, which is broadened by corneal aberrations, to create an average Gaussian distribution of ~40 μm width [24] , [25] . Next, the field was propagated down the medium, plane by plane, where every step was of 0.13 μm length. In order to test how robust was our simulation procedure, we introduced fluctuations in several parameters of the above simulation procedure (see Methods): (1) Müller cells in vivo do not appear as straight ‘nail-like’ structure, as illustrated in Fig. 1a , but rather show some bending. We use 20 random bending realizations and derive for each its wavelength properties as a wave-guiding element. (2) Perturbations were added randomly up to 5% of the cell’s width [15] in order to simulate the uneven boundaries and undulations of the cells. (3) We also added random perturbations to the cell’s refractive indices and its extracellular vicinity [26] , on a scale of 1 μm and 5–15% of the local refractive index difference between the cell and its surrounding (see Methods). The results of the simulations are robust ( Supplementary Fig. 2 ), and show that Müller cells efficiency as light guides varies with wavelength. Representative light distributions, propagating through a Müller cell for blue (430 nm) and green-yellow (560 nm) wavelengths can be seen in Fig. 1c,d respectively. The maximum output intensity of the green–yellow light distribution is nearly twice the corresponding blue light maximum ( Fig. 1c,d ; bottom). We carried out light propagation analysis through Müller cells in the human parafoveal retina for 25 distinct wavelengths spanning the visible spectrum (400 nm–700 nm). For each output light distribution, the intensity inside a circle mask ( Fig. 1e ) was summed to obtain the transmitted intensity into the central cone. To avoid the influence of the periodic intensity along the cells ( Fig. 1c,d ) we averaged it over the last cycle. The results for the entire visible spectrum ( Fig. 1e ) show that the maximum guiding efficiency occurs for green–yellow light (560 nm). This light is concentrated onto the centre—the cone receptive field area. In contrast, violet–blue light leaks outside the Müller cells to where the surrounding rods are located. To quantify the spectral effect by Müller cells, we defined a concentration factor for light in the centre of the Müller cell M ( λ ) and in its surrounding space S ( λ ). The concentration factor is the mean intensity of guided light, normalized by the mean intensity of a uniform illumination. This quantity is a ratio between the number of photons reaching a photoreceptor by Müller cell, and the number of photons that would have reached it in a free propagation (see Supplementary Methods ). The calculated results show that light concentration is wavelength-dependent and M ( λ ) has a maximum of ~11 at 560 nm ( Fig. 2a ). This means that the number of 560 nm photons reaching a single cone is 11 times larger due to Müller cells optical effect, compared with the situation in which light incident upon the retinal surface would have propagated freely through the retina. The spectrum of light transmitted by Müller cells ( Fig. 2b ) is remarkably similar to the measured spectral absorbance of human long-wavelength cones (L-cones) [27] , [28] , [29] and closely overlaps with that of medium-wavelength cones (M-cones), as shown in Fig. 2b . Interestingly, this result is consistent with the natural abundance of L- and M-cones, which accounts together for ~90% of all cones [4] , [30] . As a result of the cup-like structure (endfoot) of the most proximal portion of Müller cell, red-green light impinging upon the retina is being gathered from a large retinal region of ~20 photoreceptors, and concentrated onto a single central cone [13] . Consequently, a reduced light intensity propagates in the surrounding area, corresponding to the rods’ receptive fields. Therefore, the intensity of light in the green-red band (520–600 nm) reaching the rods is lowered by 30–40% ( Fig. 2c ), but only by 5–15% for the blue region of the spectrum ( λ <500 nm), a region to which rods are more sensitive ( Fig. 2d ). When light enters the pupil away from its centre, it reaches the retina as a tilted wavefront, rather than perpendicularly. At night time, the pupil dilates up to 8 mm, and with an average eye length of 23 mm, the maximum incidence angle with respect to the retina is ~10 0 . Therefore, we calculated also the average transmission of light in the Müller waveguide cells for light entering the eye at an incident slant of up to 10 0 , and found the same peak transmission wavelength of 560 nm ( Supplementary Fig. 3 ). 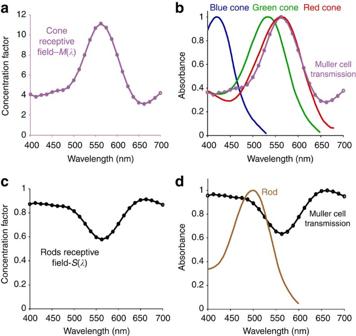Figure 2: Spectral properties of human Müller cells. (a) Light concentration factor inside a Müller cell,M(λ), exhibits a wavelength-dependent enhancement with a maximum of 11-fold for 560 nm. (b) Normalized light intensity tunnelling inside a Müller cell (purple circles) is compared with the normalized absorbance spectra of the three spectral types of human cone photoreceptors3,25,26. (c) Calculated spectrum of light leaking out of the Müller cells and illuminating the surrounding area, normalized by a uniform illumination,S(λ). The intensity is reduced by a maximum of ~40% at ~560 nm, while for blue (λ<500 nm) light the reduction is only by ~15%. (d) Normalized light intensity leaking out of Müller cells (black circles) is compared with normalized rods’ absorbance spectrum (brown)25. Figure 2: Spectral properties of human Müller cells. ( a ) Light concentration factor inside a Müller cell, M (λ), exhibits a wavelength-dependent enhancement with a maximum of 11-fold for 560 nm. ( b ) Normalized light intensity tunnelling inside a Müller cell (purple circles) is compared with the normalized absorbance spectra of the three spectral types of human cone photoreceptors [3] , [25] , [26] . ( c ) Calculated spectrum of light leaking out of the Müller cells and illuminating the surrounding area, normalized by a uniform illumination, S ( λ ). The intensity is reduced by a maximum of ~40% at ~560 nm, while for blue ( λ <500 nm) light the reduction is only by ~15%. ( d ) Normalized light intensity leaking out of Müller cells (black circles) is compared with normalized rods’ absorbance spectrum (brown) [25] . Full size image The results of the optical simulations suggest that when white light is focused upon the surface of the peripheral human retina, it is being spectrally separated by Müller cells; the green–red part of the spectrum is concentrated by up to one order of magnitude onto the cone photoreceptors and at the same time, light reaching the rods is reduced only by 5–15% for wavelengths shorter than 500 nm ( Fig. 2c,d ). Thus, Müller cells are dividing the visible spectrum in a manner that augments the cone’s light absorption, while reducing minimally light absorption by the surrounding rods. The above computational analysis was conducted for the human peripheral retina, and should also apply to other diurnal species. For nocturnal species another mechanism has been suggested, in which inverted rod nuclei act as collecting lenses, directing light onto the rod’s outer segments [31] , [32] . Experimental and computational analysis In order to examine experimentally the conclusions of the above computational analysis, we recorded the spatial and spectral distribution of light, propagating through the guinea pig retina, following by an illumination on the retinal surface, at the ganglion cells side, by a halogen light source (broad spectral source). We chose the guinea pig retina since its retinal refractive index profile and dimensions of Müller cells are known [10] , [15] . Thus, the above optical calculations can also be conducted and compared with the experimental results. A piece of a guinea pig retina was isolated from the pigment epithelium and was mounted on the stage of an inverted confocal microscope with photoreceptors facing the objective. Before recording, we identified the level of photoreceptors outer segments in order to assure that imaging was not taken within the photoreceptors layers, but at a more proximal level where Müller cells are located. For that purpose, we utilized the observation that the photoreceptors outer segments are the source of the most intense auto-fluorescence [27] , [33] within the retina, and identified the outer segment depth from the retinal surface (see Methods and Supplementary Fig. 4 ). Then, the microscope configuration was switched to record the spectral transmission of light in the retina ( Fig. 3a ). Images of transmitted light were recorded at optical sections of 5 μm thickness spanning a total of 150 μm, corresponding to the average length of Müller cells, from distal to proximal ends. We could clearly identify distinct light guiding tubes across most of the retinal depth ( Fig. 3b , in red), spanning the retina from the retinal surface down to just above the photoreceptors. The only retinal structures that fit these light-guiding tubes are the Müller cells. 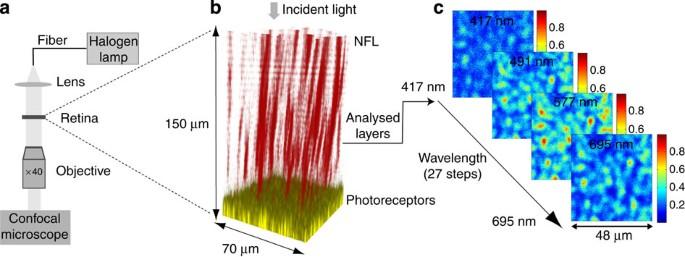Figure 3: Experimental imaging of the guinea pig retina. (a) Light from a halogen lamp is injected into an optical fibre, collimated onto the retina and imaged by a confocal microscope. (b) Light transmission through the retina is reconstructed in 3D (obtained by the microscope’szaxis stack). Distinct light tubes of high transmission—the red channel (588 nm wavelength), spanning 150 μm, from the retinal surface to just above the photoreceptor layer are observed. The yellow channel is the auto-fluorescence track, used to locate photoreceptors outer segments. For this purpose, the stack was obtained using a long working distance lens. (c) Above the level of photoreceptors, the transmitted light is imaged using the microscope’s spectral mode. The 417–695 nm range is covered by 27 distinct images at intervals of 10 nm. Four representative images (48 μm × 48 μm each) for different wavelengths (417 nm, 491 nm, 577 nm and 695 nm) are shown. Figure 3: Experimental imaging of the guinea pig retina. ( a ) Light from a halogen lamp is injected into an optical fibre, collimated onto the retina and imaged by a confocal microscope. ( b ) Light transmission through the retina is reconstructed in 3D (obtained by the microscope’s z axis stack). Distinct light tubes of high transmission—the red channel (588 nm wavelength), spanning 150 μm, from the retinal surface to just above the photoreceptor layer are observed. The yellow channel is the auto-fluorescence track, used to locate photoreceptors outer segments. For this purpose, the stack was obtained using a long working distance lens. ( c ) Above the level of photoreceptors, the transmitted light is imaged using the microscope’s spectral mode. The 417–695 nm range is covered by 27 distinct images at intervals of 10 nm. Four representative images (48 μm × 48 μm each) for different wavelengths (417 nm, 491 nm, 577 nm and 695 nm) are shown. Full size image In order to measure the spectral properties of light transmitted by Müller cells, we identified the high transmission areas (‘hot spots’) in the recorded images, taken above the photoreceptors layer ( Supplementary Fig. 5 ). These images form a set of 27 channels that covers the visible range (417–695 nm). Four representative images of four distinct spectral channels are shown in Fig. 3c . In order to quantify the spectrum of the guided light within Müller cells, we summed the pixel intensity inside the cells’ areas for the 27 monochromatic images (see three representative images of examined retina #1; Fig. 4a ). Next, we normalized the intensities of these 27 channels relative to the intrinsic halogen light source spectrum (see Methods and Supplementary Fig. 6 ). The spectral distributions of light transmitted inside 10 Müller cells ( Fig. 4b , inset) show clear enhancement for wavelengths in the red-green region of the visible spectrum in comparison to the blue-violet spectral band. The mean light intensity propagating inside these 10 Müller cells, studied in retina #1, reaches its peak at ~575 nm, and decreases towards shorter wavelengths and longer wavelengths ( Fig. 4b ). 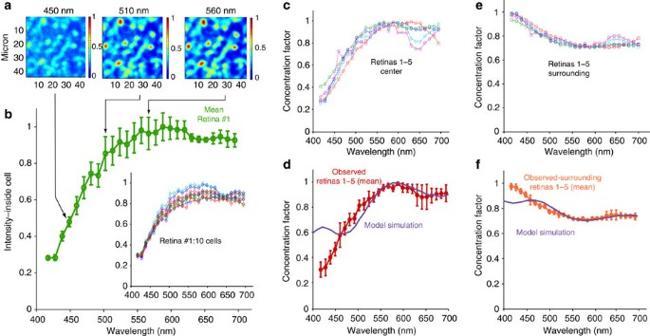Figure 4: Spectral analysis of light distribution in the guinea pig retina. (a) Twenty-seven images of transmitted light were recorded above the photoreceptors layer. Three representative images for short- (450 nm), middle- (510 nm) and long wavelengths (560 nm) are shown. The images were normalized (the sum of all pixels is equal for all images). Müller cells light tubes were located by a threshold and the 10 highest transmission cells were marked and masked. All these cells, without exception, show a higher transmission of red-green wavelengths (b, inset). (b) Mean (±s.d.) of the spectral light distribution inside Müller cells (N=10), studied in the guinea pig retina #1. Individual traces are overlaid in the inset. (c) Normalized light concentration spectra inside Müller cells (different colours), and in their surrounding areas (e) were obtained from five different retinal preparations. The mean (±s.d.) of the concentration spectra of light transmitted inside Müller cells, and in their surrounding in all studied retinas (N=5) correspond well with the concentration spectra obtained using the model simulation (purple curve) (dandf, respectively). All panels were normalized to unity at maximum. Figure 4: Spectral analysis of light distribution in the guinea pig retina. ( a ) Twenty-seven images of transmitted light were recorded above the photoreceptors layer. Three representative images for short- (450 nm), middle- (510 nm) and long wavelengths (560 nm) are shown. The images were normalized (the sum of all pixels is equal for all images). Müller cells light tubes were located by a threshold and the 10 highest transmission cells were marked and masked. All these cells, without exception, show a higher transmission of red-green wavelengths ( b , inset). ( b ) Mean (±s.d.) of the spectral light distribution inside Müller cells ( N =10), studied in the guinea pig retina #1. Individual traces are overlaid in the inset. ( c ) Normalized light concentration spectra inside Müller cells (different colours), and in their surrounding areas ( e ) were obtained from five different retinal preparations. The mean (±s.d.) of the concentration spectra of light transmitted inside Müller cells, and in their surrounding in all studied retinas ( N =5) correspond well with the concentration spectra obtained using the model simulation (purple curve) ( d and f , respectively). All panels were normalized to unity at maximum. Full size image Similar experiments were conducted in five different experimental sessions on retinas from five guinea pigs, and the resultant average spectra of light transmitted within Müller cells in these five retinas ( Fig. 4c ) show minor variations. The average spectrum of light transmitted inside Müller cells of all five guinea pigs (red curve, Fig. 4d ) shows remarkable agreement with the corresponding calculated spectrum, obtained by the optical simulation of the guinea pig retina (purple curve, Fig. 4d ). We also analysed the spectral distribution of light leakage, by measuring light outside the hot spot areas of Müller cells. The light reaching the surroundings of Müller cells also showed wavelength dependency, as illustrated by the mean spectra of the five retinas ( Fig. 4e ). The measured average spectrum (orange curve, Fig. 4f ) corresponds well with the calculated wavelength dependency of light leaking outside Müller cells as obtained by the optical simulation (purple curve, Fig. 4f ). A difference can be seen between the experimental spectra and the calculated ones within the short-wavelengths range (400–450 nm), for light transmitted inside Müller cells and for light leaking outside the cells ( Fig. 4d,f , respectively). This may result from small density fluctuations in the cells, within the path of light. These short-scale fluctuations [26] generate Rayleigh scattering of the far blue wavelengths, which cannot be simulated in the framework of beam propagation methods (BPM). It should be noted that guinea pig retina contains rods with visual pigment absorbing maximally at 500 nm and two types of cones; a short-wavelength cone (S-cone) with maximal absorption at 400 nm and a medium-wavelength cone (M-cone) with peak absorption at 530 nm (ref. 34 ). Thus, light concentration by Müller cells increases photon absorption by the distal cones, but the photon gain effect is smaller compared with the effects of Müller cells upon S-, M- and L-cones of the human equivalent (see Methods and Supplementary Fig. 7 ). Spatial alignment of cones and Müller cells To assure that the recorded light guiding tubes are directed each into a single cone photoreceptor and not randomly coupled to the photoreceptors layer, we measured the correlation between cones and light guiding tubes. For that purpose, before optical recording, cone photoreceptors were selectively labelled by FITC-PNA dye [35] (see Methods). Then, we used the multi-track mode of the confocal microscope to obtain reflection (FITC) and transmission recordings sequentially. The optical configuration was identical to the configuration we describe above for all of our experiments. However, for the transmission recording we illuminated the retina surface (ganglion cells side) with a 617 nm light-emitting diode (LED) instead of the halogen lamp, to avoid a situation in which the guided light would excite the cones’ dye and contaminate the transmission channel. We obtained stacks spanning 100 μm (50 optical slices, each 2 μm) above the photoreceptors layer. Orthogonal views of the transmission channel ( Fig. 5a ), reflection channel ( Fig. 5b ) and both channels superimposed ( Fig. 5c ) show a clear spatial association between the cones reflection and Müller cells light guiding transmission tubes. We performed quantitative analysis by thresholding both channels, at the photoreceptors layer, and comparing high-intensity areas. We found that all Müller cells were coupled to a single cone each and at least 89% of all cones were coupled to Müller cells. 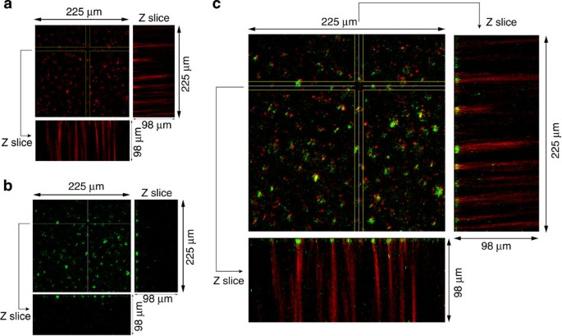Figure 5: Co-alignment between cones and Müller cells light guides. (a) Transmission channel (in red), recorded after 617 nm LED illumination from the retinal surface (ganglion cells side). (b) Reflection channel (in green), obtained by cone selective dye (FITC-PNA), and recorded by fluorescence scheme after 488 nm laser illumination from the photoreceptors side. (c) Merge of the two channels at the photoreceptors layer and in orthogonal Z slices. The Müller cells light-guiding tubes are aligned with the fluorescence green signal emitted from the labelled cones. Figure 5: Co-alignment between cones and Müller cells light guides. ( a ) Transmission channel (in red), recorded after 617 nm LED illumination from the retinal surface (ganglion cells side). ( b ) Reflection channel (in green), obtained by cone selective dye (FITC-PNA), and recorded by fluorescence scheme after 488 nm laser illumination from the photoreceptors side. ( c ) Merge of the two channels at the photoreceptors layer and in orthogonal Z slices. The Müller cells light-guiding tubes are aligned with the fluorescence green signal emitted from the labelled cones. Full size image Light absorption due to Müller cells’ spectral splitting In order to assess the effects of Müller cells spectral separation on photon absorption by cone- and rod-photoreceptors in the human parafoveal retina, we calculated light absorbance in cones’ outer segments, A Cone ( λ ) by multiplying the Müller cell’s concentration factor, M ( λ ) ( Fig. 2a ) by the normal cone absorbance profile- C ( λ ), such that A Cone ( λ )= M ( λ ) C ( λ ) ( Fig. 6a–c ). Photon absorption in rods’ outer segments A Rod ( λ ) was similarly calculated by multiplying the spectrum of light leaking outside the Müller cell into the surrounding area S ( λ ) ( Fig. 2c ), by the absorption spectrum of the rod visual pigment R ( λ ), A Rod ( λ )= S ( λ ) R ( λ ) ( Fig. 6d ). We found that the gain in photon absorption for white light impinging upon the retinal surface and propagating across the retina by the Müller cells, , showed an increase by a factor of ~7.5 for the L- and M-cones, and by a factor of ~4 for the S-cones ( Fig. 6e ). On the other hand, Müller cells’ properties cause loss in photon absorption by rods, but only by 20% ( Fig. 6e ). 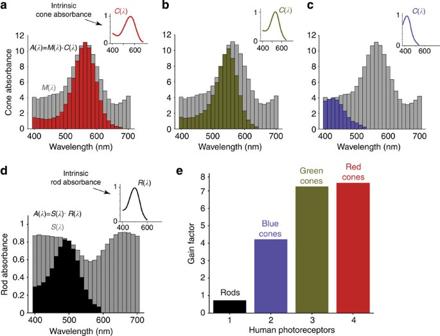Figure 6: Gain in photoreceptors light absorption in the human parafoveal retina, due to Müller cells’ spectral separation. (a–c) The gain of cones’ absorptionACone(λ)=M(λ)C(λ) (red, green and blue respectively), as derived by multiplying the Müller cell light concentration into cones,M(λ) (grey bars) by the absorption spectrum of human cones’ visual pigments (C(λ), line curves). (d) The rod absorption (black), as derived by multiplying the light spectrum leaking outside Müller cells (grey bars) by the absorption spectrum of human rod visual pigment—R(λ). (e) The total light absorption in cones is increased by Müller cells’ light concentration. The gain is highest for long-wavelength cones, slightly lower for the middle-wavelength cones, and lowest for the short-wavelength cones. Photon absorption by rods (black) is reduced by ~20%. Figure 6: Gain in photoreceptors light absorption in the human parafoveal retina, due to Müller cells’ spectral separation. ( a – c ) The gain of cones’ absorption A Cone ( λ )= M ( λ ) C ( λ ) (red, green and blue respectively), as derived by multiplying the Müller cell light concentration into cones, M (λ) (grey bars) by the absorption spectrum of human cones’ visual pigments ( C (λ), line curves). ( d ) The rod absorption (black), as derived by multiplying the light spectrum leaking outside Müller cells (grey bars) by the absorption spectrum of human rod visual pigment— R (λ). ( e ) The total light absorption in cones is increased by Müller cells’ light concentration. The gain is highest for long-wavelength cones, slightly lower for the middle-wavelength cones, and lowest for the short-wavelength cones. Photon absorption by rods (black) is reduced by ~20%. Full size image We showed here, using optical computational analysis, that white light incident upon the parafoveal retina of humans and upon the guinea pig retina, splits according to its spectral components by retinal Müller cells ( Figs 2 and 4 respectively). This was strongly supported by imaging experiments in the isolated guinea pig retina ( Fig. 4 ). The Müller cell, acting as a wavelength-dependent optical fibre, concentrates the red–green part of the spectrum inside the cells, to reach the cones, while allowing blue–violet light to leak towards the surrounding tissue, to illuminate rods. The spectrum of light transmitted through the Müller cells, derived from theoretical calculations based upon data for the human parafoveal retina, matches almost perfectly the absorption spectra of the medium- and long-wavelength human cone photoreceptors. At the same time the spectrum of light leaking outside the Müller cells matches the absorption spectrum of human rod photoreceptors. This leads to a significant gain, by a factor of ~7.5, in photon absorption by human M- and L-cones, and by a factor of ~4 for the human S-cones. This light concentration into cones is not impeding significantly light absorption in human rods' outer segments, since most of the relevant light (wavelength between 400 nm and 500 nm) leaks out from the Müller cells towards the surrounding rods ( Fig. 6 ). The computational analysis of the benefits for light transmission by human Müller cells, across the human parafoveal retina, was supported by combining computational and experimental analysis of the light guiding properties of Müller cells in the guinea pig retina. The expected effects of Müller cells in the guinea pig retina, as derived computationally from previously published refractive indices and dimensions, upon light reaching the cones and the rods, agreed almost perfectly with the experimentally derived imaging data ( Fig. 4 ). The benefits of Müller cells for cone-mediated vision in the guinea pig retina is less apparent than in human because of the different absorption spectra of guinea pig’s cone visual pigments. Nevertheless, Müller cells increased photon absorption in guinea pig M-cones by a factor of 5.1 and in S-cones by a factor of 2.1 without impeding significantly photon absorption (total reduction of 17%) in the guinea pig rods (see Supplementary Fig. 7 ). Our conclusion that retinal Müller cells, via their wavelength-dependent light guiding properties, improve photon absorption by cones, and only slightly reduce photon absorption by rods, is consistent with psychophysical tests in human observers, which are based upon rates of photon absorptions by different types of photoreceptors. In a typical Rayleigh colour match, an observer matches a yellow light (589 nm) of fixed intensity to a mixture of green (545 nm) and red (670 nm) monochromatic lights by changing the green/red intensity ratio [36] , [37] . In this well-known experiment, the green/red ratio, needed for a match to the fixed yellow light, varies between foveal viewing and peripheral viewing. This ratio decreases as the spot size is increased to cover retinal regions outside the fovea [38] . This phenomenon has been explained by several mechanisms, including intrusion of rods, pre-retinal absorption by macular pigment and changes in optical density of the cones’ visual pigments between foveal cones and parafovea cones. The separation of colours by Müller cells in the human parafovea, which has been described here, can provide another simple mechanism to explain this result. According to our findings, Müller cells concentrate yellow light (589 nm) incident on the peripheral retina and propagate it directly onto the cones, leading to ~10-fold enhancement of the yellow light photon flux ( Fig. 2a ). Thus, in order to preserve colour matching, the green and red intensities (545 and 670 nm) need to be increased similarly. However, the Müller cells increase the intensity of the 545 nm green light by ninefold and the 670 nm red light by only ~threefold ( Fig. 2a ). Therefore, the observer needs to change the green/red ratio in a manner that will increase the red at the expense of the green, leading to a reduction in the green/red ratio [31] . In another elegant psychophysical research [38] , human observers were asked to compare colours of monochromatic light between corneal illumination and trans-scleral illumination. One of the tests of that study compared the rod with cone excitation ratio for trans-scleral illumination compared with corneal illumination. It was reported that with trans-scleral illumination the rod to cone excitation ratio increased compared with the situation with corneal illumination. This observation is also consistent with our findings on the role of Müller cells in determining photon fluxes reaching the photoreceptors layer. With trans-scleral illumination, light reaches cones and rods equally, while with corneal illumination the Müller cells concentrate light towards the cones and at the same time reduce light reaching the rods, causing a decrease in rod to cone excitation ratio ( Fig. 6 ). The findings presented here indicate that the spectral separation of light by Müller cells provides a mechanism to improve cone-mediated day vision, with minimal interference with rod-mediated night vision. This is achieved by wavelength sorting of incident light by the Müller cells. Light of relevant wavelengths for cone visual pigments is directed towards the cones, while light of wavelengths more suitable for rod vision is allowed to leak outside the Müller cells towards the surrounding rods. This is a novel mechanism that needs to be considered when visual phenomena concerning cone- and rod-mediated vision are analysed. Simulated light propagation by retinal Müller cells The refractive indices of Müller cells are higher than those of their surrounding throughout the retina’s depth [10] , [11] and therefore the cells can be regarded as natural optical fibres [17] , [23] , [24] . The refractive index profile and the cell’s structure determine the efficiency of light guiding for the various wavelengths. Therefore, we first reconstructed the refractive index profile of the Müller cell and its surrounding as a function of retinal depth as can be seen in Supplementary Fig. 1a,b , using Müller cells characteristic dimensions [10] , [15] . Light passage through the retinal volume was derived using the wave equation (Helmholtz equation). The most universal method for solving the Helmholtz wave equation for a complex refractive index profiles is the FFT BPM, which is also called the split-step BPM. The method [18] , [19] , [39] is based on discretization of the continuous refractive index profile distribution. This method proved to be a very accurate, stable and in most cases efficient, for describing a variety of problems within the framework of waveguide beam propagation. The initial point of the algorithm is Helmholtz equation. When changes in the refractive index profile are moderate, the forward transmitted power is dominant. The corresponding electromagnetic field can be written as Here n and n 0 are the refractive indices of the cell and its surrounding respectively. This last assumption is also significant for the reason that it confines the algorithm to be a norm-conservative, namely the total power is conserved during propagation. The first-order numerical solution is known as the FFT-BPM: where , h is an infinitesimal propagation step in the z direction (Δ z ). k =2π/λ, is the wave number, is the two-dimensional Fourier transform and operator A f is the A operator representation in Fourier space. The method has a local error of O (ΔZ 2 ) and a global error O (ΔZ), which is very small since we used Δ z ≪ 1. A characteristic spatial intensity distribution output from a single Müller cell can be seen in Supplementary Fig. 1c for a 560 nm monochromatic light. Robustness of computational analysis We made a thorough analysis to examine how robust are the Müller cells’ spectral transmission properties. For that purpose, we added random bending of the Müller cell’s longitudinal axis. We defined our test cluster to consist of 20 different cell realizations, which were created by random axis bending ( Supplementary Fig. 2a ). We also added random perturbations on the cell’s radius on a scale of 5% of its local diameter ( Supplementary Fig. 2b ), and random perturbations to the refractive index profile, on a scale of 1 μm and ~5% of the local refractive index difference between the cell and its surrounding ( Supplementary Fig. 2c ). Higher perturbations of ~15% produced similar transmission spectrum. The normalized output intensity as a function of wavelength for the 20 cell realizations, each with independent perturbations, can be seen in Supplementary Fig. 2d . The mean±s.d. spectrum, derived from the 20 individual spectra, shows a peak transmission at the green part of the spectrum of ~560 nm ( Supplementary Fig. 2e ). These results indicate that the optical simulation of Müller cells is robust even for different bending and fluctuations in the cell’s width and index of refraction. For the illumination scheme we first generated a characteristic pupil by a circle mask and factorized it by wave fronts (phases) from typical corneal aberrations. Then, we calculated the diffraction pattern of the pupil (Fraunhofer diffraction). This calculated illumination pattern is identical to other illumination schemes obtained analytically, and generates a Gaussian distribution of ~40 μm width [4] . We also tested the spectral transmisssion obtained after using a tilted illumination, averaged up to a maximum of ~10° incidence angle on the retina (compatible with the maximal dilated pupil width of 8 mm). These results also show the same peak transmission wavelength of ~560 nm ( Supplementary Fig. 3d ). We also applied our algorithm to cones and found it to match perfectly previous results for light propagation along these cells [23] , [40] , [41] , [42] , which were obtained and examined by other methods such as coupled mode theory [22] , [43] , [44] , [45] . Animals and retina preparation All experiments were carried out according to the statement of ‘The Association for Research in Vision and Ophthalmology‘, and according to institutional guidelines. Male adult guinea pigs (500–700 g) were killed by an overdose (150 mg per kg) of sodium pentobarbital administered intraperitoneally. Freshly enucleated eyes were isolated, washed twice in a PBS and circumferentially dissected posterior to the ora serrata. Anterior segment and vitreous were carefully removed. The resulting eyecup-retina preparation was cut into 5 × 5 mm 2 segments. The retina was carefully separated from the eyecup using 30-G needles and flattened on a 0.17-mm-thick cover glass. Spectral recording of transmitted light A fresh retinal preparation was mounted on the stage of an inverted meta-confocal microscope (LSM 510 Meta; Zeiss, Germany), with photoreceptors surface facing the objective. Halogen lamp light, transmitted through an optical fibre, was collimated onto the vitreal retinal surface. The transmitted light emanating from the retina was captured through the objective. A × 40 oil immersion lens of NA=1.3 (Zeiss, Germany) was used throughout the experiments, unless indicated otherwise. For each field, the level of photoreceptors outer segments was identified before recording. This was done without the use of exogenous dyes in order to avoid any artifacts resulting from exogenous labelling. For this aim, we utilized the ‘auto-fluorescence’ nature of photoreceptor outer segments [33] , as illustrated in Supplementary Fig. 4 (excitation of 488 nm and emission of 502 nm). Following the identification of the level of photoreceptors outer segments, the microscope configuration was switched to record the spectral transmission of light in the retina. Images of transmitted light were recorded at optical sections of 5 μm thickness spanning up to 50 μm above the last auto-fluorescent section. This was done in order to validate that the recorded optical sections are proximal to the level of outer nuclear layer. For each optical section, 27 distinct spectra were obtained at intervals of 10 nm steps covering a 417–695 nm wavelengths range, using the ‘lambda mode’ of the LSM510 Meta microscope. 3D reconstruction of the light path in the retina To allow inspection of the retina at distant optical slices and in order to facilitate 3D spatial reconstruction of the light tunnelling in the retina, a × 40 lens of a NA=0.75 (Zeiss, Germany), with working distance of 0.71 mm was used (see Supplementary Data 1 ). Images obtained using such procedure served only for 3D reconstruction of light pathway, and not for spectral analysis. Optical slices spanning a ~150 μm stack of retinal volume were recorded. 3D images of the obtained stack were generated using IMARIS software (Bitplane, CT, USA). Alignment of cones and Müller cells light guides In the next sections we describe the materials and method we used for labelling the cones in the guinea pig retina, and then we describe the optical scheme for observing the alignment of cones with Müller cells light tubes. In vivo labelling of guinea pig cone photoreceptors Following anaesthesia with a mixture of ketamine 100 mg per kg + xylazine 30 mg per kg, we selectively labelled cone photoreceptors using a modified version of a previously described method [11] . In this modified version, NanoFil sub-microliter injection system with UMP-III microsyringe pump (World Precision Instruments, USA) facilitated precise and smooth injection of small dye volumes into the guinea pig vitreous humour. The system was attached to a blunt 34-G needle and preloaded with 0.5% solution of FITC-PNA in PBS (Sigma Aldrich). 0.4% Localin drops were applied and the pupils were dilated with 2.5% phenylephrine hydrochloride. At 1.5 mm behind the limbus a hole was produced using a 33-G sharp needle, and a 34-G blunt needle, connected to the NanoFil system, was inserted through this hole into the midvitreous cavity. We injected 10 μl of 0.5% FITC-PNA, retained the needle for 10 s in the vitreal cavity following injection before drawing it out, and allowed the dye to diffuse for 30 min. Thereafter, the guinea pig was killed by anaesthetic overdose. The eyes were removed and retina dissected as described above. Topographic relationship between cones and transmitted light We labelled the cone photoreceptors with FITC-PNA in vivo as described above and used the multi-track mode of the LSM 510 Meta-Confocal microscope to obtain transmission and reflection (FITC) channels sequentially. The optical configuration was identical to the configuration in all of our experiments. However, for the purpose of this experiment we used a 617 nm LED light instead of the halogen lamp to avoid a situation in which the guided light will excite the cones’ dye and contaminate the transmission channel. We also used a × 40 lens of a NA=0.75 (Zeiss, Germany) to gain deep visual field. We obtained and analysed stacks spanning 100 μm (50 optical slices, each 2 μm) above the photoreceptors layers. Spectral analysis We carried out a thorough analysis of the recorded images in order to quantify the variation of light transmission in Müller cells as a function of wavelength. The images were obtained from the retinal volume as described above (in the section ‘Spectral recording of transmitted light’). The first step was the identification of cells’ positions and inner areas using a threshold value. As a result of minor bending of the Müller cells bodies across the retina, each optical slice was composed of small intensity variations. These were generated by a small angle between the cell’s orientation and the microscope axis. Therefore, the 10 most-intense cells were marked as a mask to be analysed ( Supplementary Fig. 5 ). Each cell’s mask was applied to the 27 images, corresponding to the entire visible spectrum. The purpose of defining the brightest ten regions in each layer separately was to form a blind test: if these regions had not been continuous from layer to layer, then they were not the hallmark of light guides. The fact that they could be clearly seen across the entire retina is a significant support for the claim that Müller cells lead the light from end to end. Normalization of transmitted light In order to obtain a reliable assessment of the effects of Müller cells upon light transfer across the retina, the light reaching the photoreceptors in the distal retina needs to be normalized relative to the light incident upon the retinal surface at the ganglion cells side. The standard normalization that we used, suiting any broad spectral light source, is very commonly used in spectral measurements. It is important to emphasize that this normalization scheme enables any spectral analysis to be independent of the light source as well as the transmission optics, such as lenses or fibre optics, and detectors, such as photomultiplier tubes or CCDs. It essentially neutralizes the spectral responsivity of all of these components, as if the light source was a perfect white light (flat spectrum). In principle, this procedure derives the weights needed to transform a given spectrum of light into a flat spectrum. This transformation is used for light output based on the given light input and supplies the information of how much of each wavelength has been transmitted to the locus of measurement relative to the original intensity. We use several times the term ‘total intensity of an image’, defined as the sum over all pixels in the image. Scheme input . The microscope ‘lambda mode’ data set includes 27 images ( A 1 , A 2 , … A 27 ). Each image is a photograph taken within a narrow spectral band (11 nm). The images are spanning the visible spectrum in 27 steps ( Supplementary Fig. 6a ). Each image has different total intensity, dependent on the light source spectrum. Scheme output . New set of 27 images, where the total intensity for all images is equal. Normalization proceeds in three steps: 1 Calculate the total intensity of each image (sum over all pixels) in the original set to obtain I 1 , I 2 ,... I 27 . 2 Find the maximum intensity in the original set of 27 intensities, I max . 3 Multiply each image by the normalization weight ( I max / I i ) to derive a new set of images: The highest intensity image is multiplied by I max / I max =1, and will not be affected. All other images will be multiplied by a factor that is larger than one. As a result, we obtain a new set of images ( ) where the total intensity for all images is equal, that is, the sum of all pixels is equal in all images. This is equivalent to the situation in which a white light (perfect flat spectrum) is used for illumination. The only requirement from the source is that it provides photons in all wavelengths and it does not possess abrupt spectral changes. Therefore, we used a standard halogen lamp, possessing a black body spectrum. This light source was transmitted by a multimode, wide-band optical fibre (THORLABS FT400UMT) and recorded by the microscope lambda mode without any tissue, only with a microscope slide ( Supplementary Fig. 6a ). To obtain the spectrum of the halogen lamp and fibre we calculated the total intensity for each of the 27 images, step #1 of the scheme ( Supplementary Fig. 6b ). We applied steps #2 and #3 over this set of images and obtained a flat spectrum ( Supplementary Fig. 6c ). Any spectral recording of transmitted light, at any level within the retina, was normalized by using the normalization weights ( I max / I i ) to obtain a new set of equal intensity images ( Supplementary Fig. 6d ). This normalized set enabled obtaining the spectral transmission inside Müller cells ( Supplementary Fig. 6e ), independent of the source spectrum and the microscope responsivity (microscope PMT’s). Gain in photon absorption by guinea pig’s photoreceptors In order to calculate the effects of Müller cells light guiding properties upon photon absorption in the guinea pig photoreceptors, we compared the spectra of light transmitted by the Müller cells onto cones and of light leaking out of the Müller cells to surrounding rods, with the absorption spectra of guinea pig S- and M-cones ( Supplementary Fig. 7a ) and rods ( Supplementary Fig. 7b ). We multiplied the spectrum of each type of photoreceptor by the appropriate light spectrum to derive the gain (or loss) in photon absorption by that photoreceptor type due to the wave-guiding properties of the Müller cells ( Supplementary Fig. 7c ). The results show a total gain of 3.6 for the S-cones, 4.7 for the M-cone and 0.85 (a loss of 15%) for the rods. We also calculated the photon absorption gain using the experimentally derived spectra of light transmitted within Müller cells, and of light leaking outside the Müller cells. Therefore, we repeated the same calculations by comparing the absorption spectra of guinea pig’s photoreceptors to the experimental spectra ( Supplementary Fig. 7d–f ). This calculation ( Supplementary Fig. 7f ) gave slightly different gain value; 2.1 for S-cones, 5.1 for M-cones and 0.83 (a 17% reduction) for rods. The theoretical and experimental gain factors are similar, but not identical. We believe that the experimental values better describe the real in vivo situation. To conclude, also for the guinea pig retina, Müller cells increase photon flux reaching the cones compared with the situation where Müller cells were not behaving as wave-guides, but the effect is smaller than in the human equivalent. Spectral analysis in other tissues As an experimental control, dedicated to assure that the above spectral properties are unique to the retina, we examined the spatio-spectral distribution in another tissue, a small intestine of the mouse. We used the same halogen lamp, optical fibre and microscope configuration, as well as the same normalization scheme described above. Notably, we obtained images ( Supplementary Fig. 8a ) that bear no similarity to the images recorded from the retina, as well as a different spectral distribution ( Supplementary Fig. 8b ). The latter was obtained in the same spectral analysis scheme applied to the retina. How to cite this article: Labin, A. M. et al . Müller cells separate between wavelengths to improve day vision with minimal effect upon night vision. Nat. Commun. 5:4319 doi: 10.1038/ncomms5319 (2014).